Mutations in theGabrb1gene promote alcohol consumption through increased tonic inhibition Alcohol dependence is a common, complex and debilitating disorder with genetic and environmental influences. Here we show that alcohol consumption increases following mutations to the γ-aminobutyric acid A receptor (GABA A R) β1 subunit gene ( Gabrb1 ). Using N -ethyl- N -nitrosourea mutagenesis on an alcohol-averse background (F1 BALB/cAnN x C3H/HeH), we develop a mouse model exhibiting strong heritable preference for ethanol resulting from a dominant mutation (L285R) in Gabrb1 . The mutation causes spontaneous GABA ion channel opening and increases GABA sensitivity of recombinant GABA A Rs, coupled to increased tonic currents in the nucleus accumbens, a region long-associated with alcohol reward. Mutant mice work harder to obtain ethanol, and are more sensitive to alcohol intoxication. Another spontaneous mutation (P228H) in Gabrb1 also causes high ethanol consumption accompanied by spontaneous GABA ion channel opening and increased accumbal tonic current. Our results provide a new and important link between GABA A R function and increased alcohol consumption that could underlie some forms of alcohol abuse. Our understanding of the genetic and molecular basis of alcohol dependence is incomplete. Alcohol abuse has long been associated with facilitation of neurotransmission mediated by the brain’s major inhibitory transmitter, GABA, acting via GABA A receptors (GABA A Rs). Recently, a locus within human chromosome 4, containing GABA A R subunit genes encoding α2, α4, β1 and γ1 subunits has been associated with alcohol dependence in humans [1] , [2] , [3] , [4] , [5] , [6] , [7] . In particular, haplotypic variations in the GABRA2 gene encoding the α2 subunit have been repeatedly linked with alcohol dependence [2] , [8] , [9] , [10] . However, the neurobiological basis by which genetic variation translates into alcohol abuse is largely unknown. Ionotropic GABA A Rs are pentameric ligand-gated ion channels, drawn from a family of 19 proteins, which underpins the expression of ~20–30 neuronal GABA A R isoforms [11] . These receptors have distinct physiological and pharmacological properties, are heterogeneously expressed in the mammalian CNS and as a consequence can differentially influence behavioural phenotypes [12] , [13] . Synaptic GABA A Rs mediate phasic inhibition, whereas extrasynaptic GABA A Rs are activated by ambient concentrations of GABA and mediate a tonic form of inhibition. Recent evidence has suggested roles for both forms of GABAergic transmission in the neurobiology of addiction [14] , [15] , [16] , [17] . With regard to ethanol, both consumption and preference are reduced following disruption of GABA-mediated tonic inhibition in δ subunit knock-out (δ −/− ) mice [18] and a similar impact on ethanol drinking was achieved by RNAi-induced suppression of either α4 (a subunit partner of the δ subunit) or δ subunit expression in the rodent nucleus accumbens (NAc) [17] , [18] . The reduced ethanol self-administration appeared to be a consequence of the altered reinforcing properties of the drug [17] , [18] . These actions on ethanol drinking and self-administration appear to be specific to the activity of α4βδ receptors and not a general effect on manipulating GABAergic activity in the NAc, as no differences in ethanol self-administration have been found in α2 −/− or α5 −/− mice [19] , [20] , when compared with wild-type (WT) counterparts. It has been suggested that ethanol may exert a direct action on δ-GABA A Rs to enhance their function, which might account for the rodent self-administration data. However, whether ethanol exerts such direct effects is controversial [21] , [22] , [23] , [24] . An alternative interpretation of the behavioural data posits that the activity of NAc extrasynaptic GABA A Rs influences the activity of neural circuits underlying certain addictive behaviours such as the desire for alcohol. We were able to explore this possibility by exploiting the availability of two novel mutant mouse lines in which single point mutations in GABA A R β1 subunits have occurred. The first line was identified through a phenotype-driven N -ethyl- N -nitrosourea (ENU) mutagenesis screen [25] , [26] for alcohol-preferring mice, whereas the second was a spontaneous mutation identified using a genotype-driven approach [27] . Both mutant mouse lines display increased alcohol consumption and self-administration, and are characterized by GABA channels that can open spontaneously, promoting an increased tonic inhibition in NAc medium spiny neurons (MSNs). These findings strongly suggest that the large tonic conductance of MSNs contributes to the increased preference and intake of ethanol by Gabrb1 +/L285R and Gabrb1 +/ P228H mice. These data reveal a novel link between GABA A R function and increased alcohol consumption that could lead to a better understanding of some forms of alcohol abuse. Alcohol-preferring mouse strains We identified two dominant mutations in Gabrb1 that induced a phenotypic switch from alcohol aversion to a sustained, strongly heritable alcohol preference. One mutation was generated through phenotype-driven random ENU mutagenesis [25] , [26] ( Gabrb1 L285R ), whereas the other was a spontaneous mutation ( Gabrb1 P228H ) identified through gene-driven screening of a DNA/sperm archive [27] . Both lines showed highly penetrant ethanol preference throughout over eight and five backcross generations, respectively. An ENU-induced Gabrb1 mutation confers alcohol preference : Alcohol-averse male BALB/cAnN mice were exposed to ENU [25] and crossed to WT C3H/HeH females. G1 progeny ( n =1,047) were screened in a two-bottle choice test for preference for 10% ( v / v ) ethanol with mice showing ethanol preference backcrossed to C3H/HeH to test heritability. The ENU-induced mutation was localized to a region on mouse chromosome 5 (71.45–73.05 Mb), syntenic with a region on human chromosome 4, containing 11 genes including Gabra4 and Gabrb1 ( Supplementary Fig. S1 ). Sequencing identified just one mutation in the β1 subunit ( Gabrb1 exon 8), a leucine-to-arginine exchange (L285R) in the highly conserved third transmembrane domain (M3), near the M2–M3 linker ( Supplementary Fig. S2A ), an important area for GABA receptor activation and ion channel gating. The mutation was absent in both parental strains. A spontaneous Gabrb1 mutation confers alcohol preference : To determine whether other Gabrb1 mutations modified alcohol drinking, we screened a DNA library containing ~10,000 unique samples from ENU mutagenized male mice (F1 C57BL/6JxC3H/HeH) and identified one sample carrying a non-synonymous proline-to-histidine mutation (P228H) within M1 of the β1 subunit. This proline is highly conserved in GABA A Rs from various species ( Supplementary Fig. S2B ). While absent in both background strains, the mutation occurred in the non-ENU mutagenized C3H DNA strand and therefore had arisen spontaneously. Significantly, as with Gabrb1 +/L285R above, Gabrb1 +/P228H mutants displayed a heritable ethanol preference ( Supplementary Fig. S3 ). Gabrb1 +/L285R mutant mice were significantly smaller than WT ( P <0.0001; Supplementary Fig. S4 ). A similar but less pronounced size difference was also observed in Gabrb1 +/P228H mutant mice. Both mutant lines exhibited complete female infertility characterized by underdeveloped corpus luteii . Consequently, we could only study heterozygotes ( Gabrb1 +/L285R and Gabrb1 +/P228H ) and their corresponding WT mice. Reduced body size and impaired fertility most likely reflect hypothalamic–pituitary axis endocrine deficiency and so analysis of anterior pituitary hormone content was performed. This demonstrated that carriage of either mutant Gabrb1 allele ( Gabrb1 L285R or Gabrb1 P228H ) was associated with significant hypothalamic–pituitary axis dysfunction ( Supplementary Tables S1 and S2 ). Mutant mice displayed a significant preference for ethanol ( Gabrb1 +/L285R : Fig. 1a,b ; Gabrb1 +/P228H : Supplementary Fig. S3 ), but not for similarly presented sucrose, saccharin or quinine solutions, suggesting taste or calorific requirements were not driving alcohol preference ( Supplementary Table S3 ). Furthermore, all mice consumed similar daily fluid volumes, despite Gabrb1 +/L285R and, to a lesser extent, Gabrb1 +/P228H mutant mice possessing lower body weights ( Supplementary Fig. S4 ). The co-segregation of both alcohol preference and body weight traits were observed throughout all eight (for Gabrb1 +/L285R ) and five ( Gabrb1 +/P228H ) generations studied, being present in 123/130 (93%) of Gabrb1 +/L285R mice, effectively excluding the possibility of separate mutations causing these components. 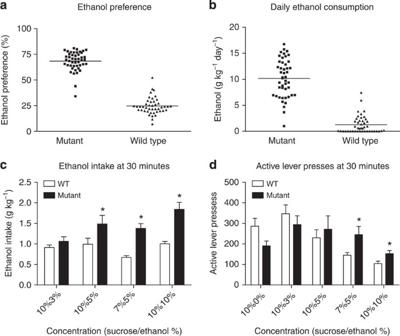Figure 1: Alcohol consumption and behavioural phenotype of Gabrb1+/L285. (a) Ethanol (10%v/v) preference of maleGabrb1+/L285(mean=68.37%, 95% CI: 65.61–71.13,n=46) and WT littermates (24.67%, 22.20–27.13,n=44;t-testP<0.0001). (b) Daily ethanol consumption (g per kg body weight): maleGabrb1+/L285(10.16, 95% CI: 9.08–11.25,n=46); WT littermates (1.24, 0.71–1.75;t-testP<0.0001,n=44). (c) Amounts of ethanol earned in operant tests (g per kg body weight±s.e.m.). *P<0.05 (n=8 per group, ANOVA plus Bonferronipost hoctest). (d) Numbers of lever presses±s.e.m. over 30 min by WT and mutant mice on a fixed ratio 4 (FR4) schedule for sucrose–ethanol reinforcers. Note increased number of lever presses for mutants at reinforcer mixtures of 7% sucrose/5% ethanol and 10% sucrose/10% ethanol (n=8/group). *P<0.05, ANOVA plus Bonferronipost hoctest. Figure 1: Alcohol consumption and behavioural phenotype of Gabrb1 +/L285 . ( a ) Ethanol (10% v / v ) preference of male Gabrb1 +/L285 (mean=68.37%, 95% CI: 65.61–71.13, n =46) and WT littermates (24.67%, 22.20–27.13, n =44; t -test P <0.0001). ( b ) Daily ethanol consumption (g per kg body weight): male Gabrb1 +/L285 (10.16, 95% CI: 9.08–11.25, n =46); WT littermates (1.24, 0.71–1.75; t -test P <0.0001, n =44). ( c ) Amounts of ethanol earned in operant tests (g per kg body weight±s.e.m.). * P <0.05 ( n =8 per group, ANOVA plus Bonferroni post hoc test). ( d ) Numbers of lever presses±s.e.m. over 30 min by WT and mutant mice on a fixed ratio 4 (FR4) schedule for sucrose–ethanol reinforcers. Note increased number of lever presses for mutants at reinforcer mixtures of 7% sucrose/5% ethanol and 10% sucrose/10% ethanol ( n =8/group). * P <0.05, ANOVA plus Bonferroni post hoc test. Full size image Gabrb1 L285R and alcohol-seeking behaviour The motivation for Gabrb1 +/L285R mice to obtain alcohol was assessed using operant self-administration of fluid coupled with a sucrose-fading technique [19] , [20] . Self-administration of ethanol over 1 h caused ataxia, consistent with alcohol intoxication ( Supplementary Fig. S5A ). To determine whether the features of intoxication observed in mutant mice during the 1 h operant sessions were due to increased intake or a heightened sensitivity to alcohol, WT and mutant mice were given a standard body-weight-adjusted dose of ethanol and tested for the presence of ataxia on the rotarod (ethanol 3 g per kg) and loss of righting reflex (ethanol 3.5 g per kg; Supplementary Fig. S5 ). Although study groups were relatively small ( n =7–8), limiting statistical power, there was a strong tendency for the mutant mice to be more impaired than the WT mice (two-way ANOVA, main effect of genotype: F (1,13)=4.46; P =0.05), and to recover more slowly (two-way ANOVA, time point*genotype interaction: F (1,13)=1.76; P =0.08). Genotype did not affect the rate of loss of righting reflex, but there was a trend towards a more rapid recovery in WT mice (806±140 versus 1466±448 s (mean±s.e.m. ); t -test, t =1.41; P <0.1). As neither the peak, nor time course of blood or brain alcohol levels differed significantly between mutant and WT mice following ethanol administration ( Supplementary Fig. S6 ), these data suggest an increased sensitivity of Gabrb1 +/L285R mice to the ataxic effects of ethanol ( Supplementary Figs S5B,C and S6 ). To ensure ataxia did not affect performance, we analysed only the first 30 min of each operant self-administration session. Although rates of lever pressing declined with lower sucrose and higher ethanol concentrations ( P <0.001, two-way ANOVA n =8 per group), these were still higher with 7/5% and 10/10% v / v sucrose/ethanol ( Fig. 1c,d ) in Gabrb1 +/L285R mice compared with WT ( P <0.01, two-way ANOVA n =8 per group). Above 5% v / v ethanol, mutant mice worked harder to obtain ethanol, irrespective of the sucrose concentration, tending towards lower lever-pressing rates for unadulterated sucrose ( P <0.1, two-way ANOVA n =8 per group). Thus, the Gabrb1 L285R mutation is specific in affecting the motivation to consume alcohol. Consistent with higher response rates, inter-response times (IRTs) were significantly shorter in the mutant mice ( Supplementary Fig. S7 ). In order to obtain information on patterns of responding within a session, we analysed the pattern of IRTs within sessions. Interestingly, WT mice showed increases in IRTs as the session progressed, consistent with them satiating on alcohol. In contrast, the Gabrb1 +/L285R mice maintained their shorter IRTs ( Supplementary Fig. S7 ). This pattern suggests that, in comparison with the WTs, their desire for alcohol decreased more slowly as they consumed alcohol. Following the tests of alcohol self-administration, the mice were tested over two sessions in extinction (that is, lever pressing no longer resulted in fluid presentation). Their response rates declined when alcohol was no longer delivered following lever presses. The higher response rates maintained by Gabrb1 +/L285R mice during extinction sessions ( Supplementary Fig. S8 ) were not significant, suggesting that there were no major differences in motivation to obtain ethanol under deprivation conditions. However, mice could not consume ethanol during extinction sessions and so any differences in rate of satiation to ethanol would not influence responding. Mutant GABA A R β1 subunits increase NAc tonic inhibition The NAc is an important brain region for understanding the neurobiology of reward and addiction. Implicating GABA A Rs, specific suppression of either the GABA A R α4 or δ subunits in the NAc decreases both ethanol consumption and preference in rats [16] , [17] . We therefore determined how the β1 mutations affected GABA A R function in NAc slices. Whole-cell voltage-clamp (–60 mV) of Gabrb1 +/L285R NAc core MSNs revealed greater membrane current noise (root mean square (RMS)) and holding currents than for WT ( Table 1 ). These effects were GABA A R-mediated as the receptor antagonist bicuculline (30 μM) induced an approximately sixfold greater outward current and a reduction in RMS for Gabrb1 +/L285R than for WT MSNs ( Table 1 , Fig. 2a,c ). Table 1 NAc tonic conductance. 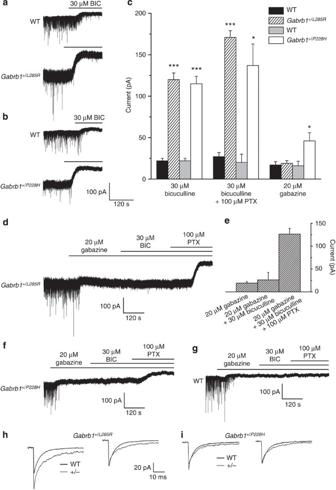Figure 2: β1 mutations influence tonic and phasic inhibition of MSNs. Whole-cell recordings from accumbal MSNs ofGabrb1+/L285R(a),Gabrb1+/P228H(b) and WT littermates. Note for bothGabrb1+/L285RandGabrb1+/P228HMSNs the larger outward currents produced by bicuculline (30 μM). Scale bars apply to bothaandb. (c) Outward currents induced by bicuculline (30 μM), gabazine (20 μM) and picrotoxin (PTX, 100 μM) from WT,Gabrb1+/L285RandGabrb1+/P228HMSNs (means±s.e.m.;n=3–12). (d) Whole-cell recording from aGabrb1+/L285RMSN. Gabazine (20 μM) abolishes the mIPSCs, but produces only a relatively small outward current. However, gabazine prevents the further outward current usually produced by bicuculline for this mutant, but not that produced by picrotoxin. (e) Mean outward current induced by GABAAR antagonists forGabrb1+/L285RMSNs (means ±s.e.m.;n=4). Whole-cell recordings from aGabrb1+/P228H(f) and a WT MSN (g). Gabazine (20 μM) abolishes mIPSCs, but additionally produces only a relatively small outward current for both theGabrb1+/P228Hand WT MSNs. However, for theGabrb1+/P228HMSN gabazine prevents a further outward current by subsequent bicuculline, but this antagonist does not prevent the outward current produced by picrotoxin. By contrast, for WT MSNs after gabazine both bicuculline and picrotoxin are inert. Superimposed averaged mIPSCs are shown for WT (black) andGabrb1+/L285R(h), orGabrb1+/P228H(i) MSNs (grey). Right-hand traces of each pair are normalized to the mean peak amplitude of the appropriate WT mIPSC. Note the prolonged mIPSCs forGabrb1+/L285RandGabrb1+/P228Hover WT. Scale bars apply to bothhandi. *P<0.05, ***P<0.001 (unpaired Student’st-test for mutants relative to WTs). Full size table Figure 2: β1 mutations influence tonic and phasic inhibition of MSNs. Whole-cell recordings from accumbal MSNs of Gabrb1 +/L285R ( a ), Gabrb1 +/P228H ( b ) and WT littermates. Note for both Gabrb1 +/L285R and Gabrb1 +/P228H MSNs the larger outward currents produced by bicuculline (30 μM). Scale bars apply to both a and b . ( c ) Outward currents induced by bicuculline (30 μM), gabazine (20 μM) and picrotoxin (PTX, 100 μM) from WT, Gabrb1 +/L285R and Gabrb1 +/P228H MSNs (means±s.e.m. ; n =3–12). ( d ) Whole-cell recording from a Gabrb1 +/L285R MSN. Gabazine (20 μM) abolishes the mIPSCs, but produces only a relatively small outward current. However, gabazine prevents the further outward current usually produced by bicuculline for this mutant, but not that produced by picrotoxin. ( e ) Mean outward current induced by GABA A R antagonists for Gabrb1 +/L285R MSNs (means ±s.e.m. ; n =4). Whole-cell recordings from a Gabrb1 +/P228H ( f ) and a WT MSN ( g ). Gabazine (20 μM) abolishes mIPSCs, but additionally produces only a relatively small outward current for both the Gabrb1 +/P228H and WT MSNs. However, for the Gabrb1 +/P228H MSN gabazine prevents a further outward current by subsequent bicuculline, but this antagonist does not prevent the outward current produced by picrotoxin. By contrast, for WT MSNs after gabazine both bicuculline and picrotoxin are inert. Superimposed averaged mIPSCs are shown for WT (black) and Gabrb1 +/L285R ( h ), or Gabrb1 +/P228H ( i ) MSNs (grey). Right-hand traces of each pair are normalized to the mean peak amplitude of the appropriate WT mIPSC. Note the prolonged mIPSCs for Gabrb1 +/L285R and Gabrb1 +/P228H over WT. Scale bars apply to both h and i . * P <0.05, *** P <0.001 (unpaired Student’s t -test for mutants relative to WTs). Full size image Accumbal MSNs exhibit a GABA-dependent tonic conductance mediated by extrasynaptic α4βδ receptors [28] . However, the inward current induced by the agonist THIP, at a δ-GABA A R-selective concentration (1 μM) was similar for WT and Gabrb1 +/L285R MSNs, implying that the large tonic current for Gabrb1 +/L285R was not caused by increased δ-GABA A R expression ( Table 1 ). In contrast to bicuculline (a partial negative allosteric modulator [29] , [30] , [31] ), the competitive antagonist gabazine (20 μM) only induced small outward currents in both WT and L285R MSNs ( Table 1 , Fig. 2c–e ), suggesting increased ambient levels of agonist (for example, GABA, taurine) do not cause the larger tonic current. The differential influence of GABA A R antagonists on Gabrb1 +/L285R neurons may indicate that bicuculline, but not gabazine, shuts spontaneously open mutant β1 GABA A R channels [29] , [32] . Indeed, picrotoxin (100 μM), which is a non-competitive antagonist of GABA A R-gated chloride channels, when co-applied with bicuculline, produced an additional outward current selectively in Gabrb1 +/L285R neurons ( Table 1 ; Fig. 2c ), whereas gabazine (20 μM), which shares a common binding site with bicuculline, prevented the outward current induced by bicuculline (30 μM), but not by picrotoxin (100 μM; Table 1 , Fig. 2d,e ). Gabrb1 +/P228H MSNs also exhibited a greater membrane current noise and holding current than WT MSNs ( Table 1 ). In Gabrb1 +/P228H neurons, bicuculline (30 μM) and, to a lesser extent, gabazine (20 μM), induced larger outward currents relative to WT ( Fig. 2b,c ). In common with the β1L285R mutation, after gabazine, the co-application of picrotoxin (100 μM) to Gabrb1 +/P228H , but not to WT MSNs, induced an additional outward current ( Fig. 2f,g ). Furthermore, as for β1 L285R , gabazine prevented the additional outward current produced by bicuculline in Gabrb1 +/P228H MSNs ( Table 1 ; Fig. 2f ). Thus, Gabrb1 P228H enhanced the tonic conductance, consistent with the ability of these mutant β1 GABA A Rs to open spontaneously. β1 subunit mutations influence NAc phasic inhibition The β1 subunit mutations also affected GABA A R-mediated phasic inhibition. For Gabrb1 +/L285R and Gabrb1 +/P228H MSNs the frequency of mIPSCs was reduced and their decay times prolonged. Additionally, the mIPSC amplitude was increased for Gabrb1 +/L285R relative to WT MSNs ( Fig. 2h,i ; Table 2 ),which was associated with an increased population of large amplitude mIPSCs, exhibiting slow decays. A scatter plot revealed a cluster of large amplitude (peak amplitude >105 pA), slowly decaying (T70 >19 ms) events prevalent in Gabrb1 +/L285R MSNs constituting only 0.7% of the total number of events for WT MSNs, but 8.8% (>10-fold increase) of the Gabrb1 +/L285R MSNs ( Supplementary Fig. S9 ). Conversely, the proportion of events with a peak amplitude <105 pA and T70 <19 ms decreased from 81.7% for WT to 54.2% for the Gabrb1 +/L285R MSNs. This loss is accounted for not only by the greater percentage of events with a peak amplitude >105 pA and T70 >19 ms but, additionally, by a higher proportion of events with an amplitude >105 pA (T70 ≤19 ms) and of those with a T70 >19 ms (but pA ≤105 pA) ( Supplementary Fig. S9 ). Such events may originate from a population of mutant postsynaptic β1-GABA A Rs, with increased open probabilities compared with WT β1-GABA A Rs. Table 2 Brain slice electrophysiology: synaptic transmission. Full size table Both the L285R and the P228H mutations were associated with a reduced mIPSC frequency compared with WT counterparts ( Supplementary Table S2 ). Activation by THIP of presynaptic δ-GABA A Rs, located either on accumbal interneurons (the main source of MSN somatic input) or on neighbouring MSNs, reduces GABA release onto MSNs (mIPSC frequency, control: 1.9±0.2 Hz; +THIP 1 μM: 1.1±0.2 Hz, data presented as mean±s.e.m., n =5; P <0.05 paired t -test). Therefore, it is conceivable that pre-synaptically located spontaneously open β1-GABA A Rs either on interneurons or neighbouring MSNs would similarly influence GABA release, thereby reducing MSN mIPSC frequency. Mutant β1 subunit expression and spontaneous channel opening To explore how the β1 L285R and β1 P228H mutations affected GABA A R function, we used heterologous expression of WT and mutant recombinant GABA A Rs in HEK293 cells. Immunocytochemistry was used to assess the expression levels of myc epitope-tagged WT and mutant β1 subunits. The expression levels of β1 L285R along with α2 and γ2L subunits, including enhanced green fluorescent protein (eGFP), revealed no differences either for cell surface or overall total fluorescence ( Supplementary Fig. S10 ). Similarly, the cell surface membrane and intracellular expression levels for β1 P228H were also unaltered compared with WT β1 subunits ( Supplementary Fig. S11 ). To examine whether the β1 subunit mutations (L285R and P228H) altered GABA A R receptor physiology and pharmacology, whole-cell recording was performed on α2β1 L285R γ2 and α2β1 P228H γ2 receptors expressed in HEK293 cells. Relative to WT, both mutations reduced the maximum current density induced by saturating GABA concentrations (1 mM; Fig. 3a ). 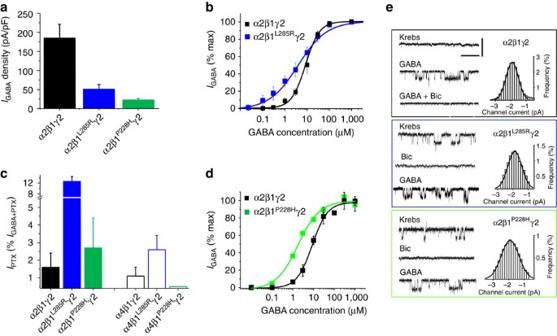Figure 3: Effects of β1L285Rand β1P228Hon recombinant GABAARs. (a) Mean maximal GABA current densities to saturating GABA concentrations for WT and mutant, α2β1γ2 receptors. (b) GABA concentration–response curves for WT and α2β1L285Rγ2 receptors. Responses are normalized to the maximum response from each cell. (c) Mean maximal outward currents produced by picrotoxin (PTX; 100 μM) for WT and mutant receptors. Values are percentages of total current (=IPTX/(IPTX+IGABA Max). (d) GABA concentration–response curves for WT and α2β1P228Hγ2 receptors, analysed as in (b). (e) Single channel currents (sampled at 50 kHz) from outside-out patches (−70 mV) of HEK293 cells expressing α2β1γ2, α2β1L285Rγ2 and α2β1P228Hγ2 receptors. Spontaneous channel activity is evident in the absence of GABA (traces labelled ‘Krebs’). Both spontaneous and GABA-activated channel openings are inhibited by bicuculline (Bic: 50 μM). Scale bars: 2 pA, 100 ms. Single channel amplitude histograms (right panels) are based on 10–30 s epochs for α2β1γ2 (activated by 10 μM GABA) and for spontaneously active α2β1L285Rγ2 and α2β1P228Hγ2. All single channel currents have mean amplitudes of approximately −1.9 pA (~27 pS). Error bars in panelsa–drepresent the mean ±s.e.m. (n=7–15 fora:n=4–6 for panelsbandd:n=6–11 forc). Figure 3: Effects of β1 L285R and β1 P228H on recombinant GABA A Rs. ( a ) Mean maximal GABA current densities to saturating GABA concentrations for WT and mutant, α2β1γ2 receptors. ( b ) GABA concentration–response curves for WT and α2β1 L285R γ2 receptors. Responses are normalized to the maximum response from each cell. ( c ) Mean maximal outward currents produced by picrotoxin (PTX; 100 μM) for WT and mutant receptors. Values are percentages of total current (= I PTX /( I PTX + I GABA Max ). ( d ) GABA concentration–response curves for WT and α2β1 P228H γ2 receptors, analysed as in ( b ). ( e ) Single channel currents (sampled at 50 kHz) from outside-out patches (−70 mV) of HEK293 cells expressing α2β1γ2, α2β1 L285R γ2 and α2β1 P228H γ2 receptors. Spontaneous channel activity is evident in the absence of GABA (traces labelled ‘Krebs’). Both spontaneous and GABA-activated channel openings are inhibited by bicuculline (Bic: 50 μM). Scale bars: 2 pA, 100 ms. Single channel amplitude histograms (right panels) are based on 10–30 s epochs for α2β1γ2 (activated by 10 μM GABA) and for spontaneously active α2β1 L285R γ2 and α2β1 P228H γ2. All single channel currents have mean amplitudes of approximately −1.9 pA (~27 pS). Error bars in panels a – d represent the mean ±s.e.m. ( n =7–15 for a : n =4–6 for panels b and d : n =6–11 for c ). Full size image As native GABA A Rs contain two β subunits and because our in vivo studies necessarily used heterozygous mice, a proportion of native GABA A Rs could comprise a mixture of WT and mutant β1 subunits. To examine the amplitudes of GABA-evoked currents under these conditions, we recreated a binomial mixture of GABA A Rs in HEK293 cells by co-expressing α2 and β1 with either β1 L285R or β1 P228H and γ2 subunits in an equimolar ratio, thereby reproducing native receptor isoforms likely to be present in heterozygotes. Assuming receptor subunit assembly proceeds according to binomial probabilities, we would expect a mixture of pentameric receptors (2α:2β:1γ) to include: WT, full mutant (both β subunits are mutated) and two forms of partial mutant receptors containing only one copy of the mutant β subunit. The maximum current densities induced by saturating concentrations of GABA (up to 1 mM) were larger for receptors containing only one copy of the mutant β subunit than those observed with full mutant receptors, and this approached that of WT receptors ( Supplementary Fig. S12 ). GABA concentration–response curves revealed that GABA potency was increased (~2–3-fold) by β1 L285R and β1 P228H ( Fig. 3b,d ; Supplementary Table S4 ). Significantly, the holding current (at −40 mV) was greater for many mutant receptor-expressing cells compared with WT ( Supplementary Table S4 ), indicative of spontaneous GABA channel activity [33] . Indeed, picrotoxin (100 μM) induced outward currents in the absence of GABA for cells expressing β1 L285R , and to a lesser extent for β1 P228H mutant receptors, reflecting spontaneous channel activity ( Fig. 3c ). The spontaneous current revealed by picrotoxin ( I PTX ) accounted for ~3–15% of the total current (= I GABA,max + I PTX ) for these mutant receptors. We also examined the level of spontaneous current for α4β1γ2 receptors, with WT or mutant β1 subunits, as an alternative isoform that may populate synaptic and/or extrasynaptic sites. Maximal current densities and holding currents exhibited greater variability for the β1 mutants compared with WT ( Supplementary Table S4 ), and α4β1 L285R γ2 exhibited a spontaneous current revealed by picrotoxin ( Fig. 3c ). To examine the gating of GABA ion channels underlying the spontaneous current, we used outside-out patches from HEK293 cells expressing α2β1γ2, α2β1 L285R γ2 or α2β1 P228H γ2 receptors ( Fig. 3e ). Spontaneous channel activity was evident with mutant receptors, but absent in WT, and abolished by the GABA antagonist, bicuculline (50 μM), acting as a negative allosteric modulator [29] in the absence of GABA. Activating WT α2β1γ2 GABA channels with 10 μM GABA induced single-channel currents that were indistinguishable from the spontaneous openings observed with the mutant receptors ( Fig. 3e ) and with only minor differences in open and shut time durations ( Supplementary Table S5 ). Overall, β1 L285R , but to a lesser extent, β1 P228H caused spontaneous channel opening and increased receptor sensitivity to GABA when co-assembled with either α2 or α4 and γ2 subunits. Given the importance of α4 and δ subunits for tonic current in NAc MSNs [16] , [17] , [28] we explored whether β1 mutants also conferred spontaneous channel activity on δ-GABA A Rs. Using HEK293 cells, β1 subunits were expressed with either α2 (co-located on same chromosome as β1, and expressed in accumbal synapses [34] ), or α4 (co-expressed in the accumbens with δ forming extrasynaptic receptors) [28] . The β1 L285R mutation increased the maximum current density to saturating GABA (300 μM) for both α2β1 L285R δ and α4β1 L285R δ receptors, compared with WT equivalents (α2/4β1δ), whereas β1 P228H did not ( Supplementary Fig. S13 ). Both β1 mutants increased GABA sensitivity by 3–5-fold at α2β1δ-GABA A Rs ( Fig. 4a , Supplementary Table S4 ), similar to the increased sensitivity for mutant α2β1γ GABA A Rs ( Fig. 3b ), but only β1 L285R affected α4β1δ receptor sensitivity to GABA ( Fig. 4b ). 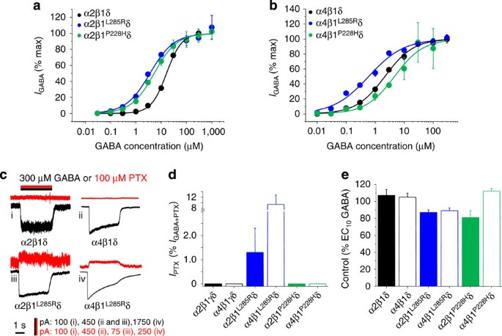Figure 4: Effects of β1L285Rand β1P228Hon δ-containing recombinant GABAARs. (a,b) GABA concentration–response curves for WT and mutant α2β1δ and α4β1δ receptors, analysed as inFig. 3b. (c) Representative membrane currents for GABA (black) or picrotoxin (red) recorded for WT and mutant (L285R) α2β1δ and α4β1δ receptors (VH=−40 mV). (d) Mean maximal outward currents after PTX (100 μM; expressed as inFig. 3c) applied in the absence of GABA for WT and mutant α2β1δ (solid bar) or α4β1δ (open bar) receptors. (e) Mean GABA responses (EC10) in the presence of 30 mM EtOH for WT and mutant receptors (Control EC10responses=100%). All error bars ina,b,danderepresent the mean ±s.e.m. (n=5–12 foraandb:n=7–12 ford:n=3–13 fore). Figure 4: Effects of β1 L285R and β1 P228H on δ-containing recombinant GABA A Rs. ( a , b ) GABA concentration–response curves for WT and mutant α2β1δ and α4β1δ receptors, analysed as in Fig. 3b . ( c ) Representative membrane currents for GABA (black) or picrotoxin (red) recorded for WT and mutant (L285R) α2β1δ and α4β1δ receptors ( V H =−40 mV). ( d ) Mean maximal outward currents after PTX (100 μM; expressed as in Fig. 3c ) applied in the absence of GABA for WT and mutant α2β1δ (solid bar) or α4β1δ (open bar) receptors. ( e ) Mean GABA responses (EC 10 ) in the presence of 30 mM EtOH for WT and mutant receptors (Control EC 10 responses=100%). All error bars in a , b , d and e represent the mean ±s.e.m. ( n =5–12 for a and b : n =7–12 for d : n =3–13 for e ). Full size image In the absence of GABA, picrotoxin (100 μM) induced outward currents only for α2/4β1 L285R δ GABA A Rs ( Fig. 4c,d ), with α2/4β1 P228H δ showing similar levels of activity to WT. Given that β1 L285R conferred substantial spontaneous activity on δ-GABA A Rs, compared with β1 P228H , the increased tonic currents recorded in MSNs of the NAc and caused by the β1 mutants are most likely due to the presence of α2/4β1 L285R γ2, α2/4β1 P228H γ2 and α2/4β1 L285R δ isoforms. Alcohol and GABA A Rs Although alcohol may directly modulate some GABA A Rs, this remains controversial [21] , [22] , [35] , [36] . Here ethanol (30–200 mM) co-applied with low concentrations (EC 10 ) of GABA did not modulate α2/α4β1γ2 GABA A Rs containing either WT or mutant β1 subunits in HEK cells ( Supplementary Table S4 ). Alcohol intoxication is associated with increased production of the endogenous neurosteroid allopregnanolone, an allosteric potentiator of GABA A Rs [35] . However, WT and β1 mutant GABA A Rs remained equally sensitive to potentiation by allopregnanolone (1 μM) and benzodiazepines (0.5 μM diazepam), and to inhibition by Zn 2+ (100 μM) or bicuculline (50 μM) ( Supplementary Figs S14 and S15 ). Similarly, neither β1 mutant when co-expressed with α2δ or α4δ subunits demonstrated sensitivity to 30 or 100 mM ethanol ( Fig. 4e ). Potentiation of αβδ GABA A R function by neurosteroids (THDOC) was also unaffected by the mutation ( Supplementary Fig. S13 ). A previous study in the dorsal striatum clearly demonstrated that acute ethanol decreased the amplitude of the electrically evoked IPSCs recorded from MSNs of young rats, but with no effect on the paired pulse ratio, suggesting a postsynaptic locus [37] . However, in our recordings from mature mouse NAc MSNs, ethanol (50 mM) had no significant effect on the spontaneous IPSCs (paired recordings n =5 neurons from 5 mice per genotype; Supplementary Fig. S16 ). Note that although there was an apparent trend for ethanol to increase the frequency of sIPSCs in the Gabrb1 +/L285R MSNs, it was not significant in this sample. In further agreement with the recombinant receptor experiments, ethanol (50 mM) had no effect on the holding current of WT or Gabrb1 +/L285R MSNs (paired recordings n =5 neurons from 5 mice per genotype; Supplementary Fig. S16 ). Thus, it is evident that the L285R and P228H mutations do not affect the co-assembly of β1 with α2/4, δ and γ2 subunits, or their pharmacological properties. ENU mutagenesis [25] of alcohol-averse BALB/cAnN mice generated a stable line carrying a non-synonymous dominant mutation in Gabrb1 (L285R) with a strong phenotypic preference for alcohol. Given that the probability of a second ENU-induced mutation within a 5-Mb region is estimated to be P <0.002 (using both a Maximum Likelihood Estimation method, adopting a Poisson model, and a Markov chain Monte Carlo method, with a Poisson Gamma model) [38] , [39] , the probability of a second functional mutation within the 1.6-Mb genomic region of interest is extremely remote and would continue to halve with each of the subsequent eight backcross generations that have been studied. This possibility has been further excluded by the absence of other exonic mutations following comparative sequencing across the candidate region. Importantly, the identification of a second, independent line with a spontaneous, non-synonymous single base-pair mutation (P228H) in the same gene that also consistently exhibits ethanol preference and similar phenotypic traits over the five backcross generations studied, provides further confirmation that the phenotype is caused by mutating Gabrb1 . Mutant and WT mice showed no differences in preference for saccharin or quinine solutions, discounting taste as a driver for high alcohol consumption by the mutants. That Gabrb1 +/L285R mice worked harder than WT to obtain alcohol compared with sucrose solutions indicates that motivation for alcohol was also not driven by calorific requirement or taste. Importantly, mutants undertook this extra work despite possessing lower body weights than their WT counterparts. The mutant mice also showed greater sensitivity to the sedative/ataxic effects of ethanol, which together with increased consumption, contributed to an increased incidence of intoxication. Previous studies in man demonstrated significant allelic association between the risk of alcohol dependence and GABRA2 and GABRB1 polymorphisms [4] , [5] , [40] , [41] , [42] . Although deleting Gabra2 in mice did not alter ethanol self-administration [19] , and human polymorphisms and mouse mutations may lack common effects on receptor function, our studies are supportive of the view that the GABA A R β1 subunit is a modifier of alcohol consumption. The NAc is associated with reward and has an important role in addiction. Our recordings from MSNs within the accumbal core revealed that the β1 subunit mutations greatly impact upon both synaptic and tonic inhibitory transmission. For Gabrb1 +/L285R and Gabrb1 +/P228H , mIPSCs were prolonged and less frequent. Given our previous demonstration that MSNs express synaptic α2-GABA A Rs [34] , the changed mIPSC kinetics suggest that β1 subunits may co-assemble with α2 and γ2 subunits at inhibitory synapses. The GABA A R-mediated tonic conductance was greatly increased in the NAc of Gabrb1 +/L285R and Gabrb1 +/P228H mice. The differential effects of GABA A R antagonists suggest that this perturbation results from spontaneous activity of mutant β1-GABA A Rs, though increased receptor sensitivity to GABA and, for Gabrb1 +/P228H , an increase in ambient GABA may also contribute. Our recombinant receptor studies indicate that mutant β1 subunits efficiently co-assemble with α and γ or δ subunits and are functionally expressed at the cell surface, with minimal effect on their pharmacological properties. Nevertheless, both β1 P228H and β1 L285R mutations increased receptor sensitivity to GABA and caused their channels to open spontaneously in the absence of GABA, particularly for L285R. Modelling the likely subunit combinations of synaptic α2- and extrasynaptic δ-containing GABA A Rs found in accumbal MSNs, we recreated recombinant equivalents of extrasynaptic (α2/4β1δ) and synaptic (α2/4β1γ2)-type receptors. Mutating the β1 subunit initiated spontaneous GABA channel opening, with β1 L285R exhibiting a greater degree of spontaneous activity, implying that both αβ1 L285R γ and αβ1 L285R δ receptors are the most significant contributors to the increased spontaneous (tonic) current in the NAc of the Gabrb1 +/L285R mouse. In comparison, β1 P228H GABA A Rs were less spontaneously active, but such activity was nevertheless clearly evident for α2β1 P228H γ2. Recombinant GABA A Rs (α2/α4β1γ2, α2/α4β1δ) incorporating either WT or mutant β1 subunits were consistently insensitive to ethanol. Similarly, neither tonic nor phasic inhibition of WT and β1 mutant MSNs was affected by ethanol. Although low ethanol concentrations (~10–30 mM) have been reported to enhance neuronal and recombinant δ-GABA A R [21] , [23] function, other studies have failed to corroborate such effects [22] , [24] , [43] , [44] , [45] . Thus, increased accumbal tonic current is associated with β1 subunit mutations leading to increased ethanol consumption, but not as a consequence of direct effects of ethanol on GABA A Rs. Notably, both ethanol preference and consumption are reduced in δ −/− mice [18] , a genetic manipulation that reduces accumbal tonic currents [28] . The importance of the tonic current for ethanol reward is emphasized by RNAi knockdown of either α4 or δ subunits in the accumbens, which reduced ethanol consumption and preference without affecting water or sucrose intake [16] , [17] . Collectively, this strongly suggests that the large tonic conductance of MSNs contributes to the increased preference and intake of alcohol by Gabrb1 +/L285R and Gabrb1 +/ P228H mice. Our study identifies GABA A Rs containing the β1 subunit as a key element in modulating alcohol consumption and suggests that spontaneous GABA channel opening and increased tonic inhibition in the accumbens are critically important factors in this debilitating behavioural phenotype that is so costly to individuals and society. Mice Mice were housed under standard conditions with a commercial diet (SDS, UK) and drinking water ad libitum . Using alcohol-averse background strains, 12-week-old male BALB/cAnN mice were exposed to ENU [25] and crossed to WT C3H/HeH females. G1 progeny ( n =1,047) were screened in a two-bottle choice test for preference for 10% ( v / v ) ethanol at age 7–12 weeks. Mice showing ethanol preference (>2.5 s.d. above a control non-mutagenized BALB/cAnN x C3H/HeH cohort) were backcrossed to 8–12-week-old C3H/HeH females to test heritability. Our study was approved by the local ethical review panels of the MRC Mammalian Genetics Unit (MRC Harwell), the University of Dundee and the University of Sussex, and complies with the UK Animal (Scientific Procedures) Act 1986. Phenotyping Male and female 7–12-week-old adult mice were singly housed with free choice of water or ethanol (3 or 10% v / v ) during two 10-day test periods. Consumption was determined by weighing the drinking bottles. The amount consumed was corrected for leakage and evaporation and expressed as grams ethanol consumed daily per kg body weight of the mice measured at the beginning of each period. Preference was calculated as the ratio of ethanol over total amount of liquid imbibed. Taste preference was determined similarly using 15 and 120 mM sucrose (caloric value), 0.25 mM and 0.4 mM saccharin (no caloric value) and 0.05 mM quinine. For self-administration of ethanol studies, animals ( n =8 group) were trained using a sucrose-fading procedure to self-administer up to 10% v / v ethanol [19] , [20] . Intoxication was scored as normal, mild ataxia or ambulatory impairment, upon removal of the animals from the operant boxes at the end of daily sessions. Mapping of ENU Mutation A genome scan was performed on 13 animals (2 G2, 11 G3) displaying high ethanol preference using 86 microsatellite markers distributed throughout the genome to differentiate DNA of BALB/cAnN or C3H/HeH origin. A further 169 animals were used to identify informative recombinants. Fine mapping with additional microsatellite markers in the candidate region was undertaken to narrow the location of the mutation. Candidate gene sequencing Exons and the exon/intron borders of twelve candidate genes were sequenced from both directions in mutant and WT mice. Oligonucleotides were designed using Ensembl v36 predictions ( http://ensembl.org ). Data were analysed with BioEdit software. Primer sequences can be found in Supplementary Table S6 . Electrophysiology and analysis of brain slice preparations Coronal slices (300 μm) containing the NAc were prepared from male Gabrb1 +/L285R , Gabrb1 +/P228H and WT littermates (age 2–5 months). As previously described [34] , slices were cut in oxygenated ice-cold maintenance solution containing (mM): 140 K gluconate, 15 Na gluconate, 4 NaCl, 10 HEPES and 0.2 EGTA (pH 7.2; 310–320 mOsm), before storage for at least 1 h at room temperature (20–23 °C) in oxygenated, extracellular solution (ECS) containing (mM): 126 NaCl, 2.95 KCl, 26 NaHCO 3 , 1.25 NaH 2 PO 4 , 2 CaCl 2 , 10 D -glucose and 2 MgCl 2 (pH 7.4; 300–310 mOsm). MSNs were identified with an Olympus BX51 microscope equipped with DIC/infrared optics. Whole-cell voltage-clamp recordings (−60 mV) were performed at 35 °C, using the ECS containing 1 μM strychnine, 2 mM kynurenic acid and 0.5 μM tetrodotoxin (TTX). Patch electrodes (3–4 MΩ) were filled with (mM): 135 CsCl, 10 HEPES, 10 EGTA, 1 CaCl 2 , 2 MgCl 2 and 2 Mg-ATP, 5 QX-314 (pH 7.2–7.3 with CsOH, 300–308 mOsm). Recordings were discarded if series resistance changed by >20%. Currents were filtered at 2 kHz (8-pole, low-pass Bessel filter) and recorded for offline analysis (DTR1205 recorder). Bicuculline methobromide, gabazine, THIP and strychnine hydrochloride were prepared as aqueous stock solutions for dilution in ECS. Picrotoxin was prepared in ECS. All drugs were obtained from Sigma-Aldrich (Poole, UK) or Tocris Bioscience (Bristol, UK). THIP and ethanol were allowed to infiltrate the slice for at least 10 min before data acquisition. Recordings were digitized (NIDQMX, National Instruments) and sampled at 10 kHz before analysis (WinEDR/WinWCP). The mIPSCs were threshold-detected (−4 pA, duration 3 ms) and visually inspected. A minimum of 50–100 mIPSCs were used for analysis, including peak amplitude, rise time (10–90%, ≤1 ms) and decay times. The decay phase of mIPSCs was best fit (98–10% of the peak amplitude) with a bi-exponential ( y ( t )= A fast e (− t / τ fast) + A slow e (− t / τ slow) ) function, where t is time, A is the amplitude and τ is the decay time constant. A weighted decay time constant ( τ w ) was calculated from the equation: τ w = τ 1 P 1 + τ 2 P 2 , where τ 1 and τ 2 are decay time constants and P 1 and P 2 the relative proportions of the decay described by each component. The mIPSC frequency was determined in 20-s bins for 2 min, detected by the rate of rise (30–50 pA ms −1 ), excluding spurious noise. The mean current and associated RMS were calculated over 102.4 ms epochs for 1 min, using a 10-kHz sampling rate. Epochs containing mIPSCs or unstable baseline were excluded. To ensure changes in the holding current reflected a drug effect, two 1-min control holding current periods (C1 and C2) were sampled and a 1-min section after drug equilibration (D). The mean holding current for C1 and C2 were pooled and the s.d. calculated. The drug effect was accepted if the absolute change in the holding current (D−C2) was greater than twice the standard deviation of the controls (C1, C2). For electrophysiological analysis of brain slice recordings all data reported represent the mean±s.e.m. of observations derived from a minimum of three animals and each determination is derived from an individual slice. Site-directed mutagenesis All point mutations in the GABA A R β subunit were introduced using Quikchange (Stratagene). Sequences of the full coding region of mutated murine cDNAs were determined by automated fluorescent sequencing. Plasmid DNAs for transfection were purified using the Hi-Speed Plasmid Midi Kit (Qiagen). Cell culture and electrophysiology HEK293 cells (ATCC, Middlesex, UK) were cultured in Dulbecco’s modified Eagle’s medium with 10% v / v fetal calf serum, 2 mM glutamine, 100 units per ml penicillin G and 100 mg ml −1 streptomycin at 37 °C in 95% air/5% CO 2 . Cells were transiently transfected by calcium phosphate co-precipitation using 1 μg of each plasmid DNA encoding for α2, α4, β1, δ or γ2 and 0.5 μg Enhanced Green Fluorescent Protein (GFP; Clontech) and used for electrophysiology after 20 h. Whole-cell currents were recorded at room temperature (20–22 °C) from single HEK293 cells voltage clamped at −40 mV, using an Axopatch 200B amplifier (Molecular Devices, USA). Patch electrodes (3–5 MΩ) contained (mM): 144 KCl, 2 MgCl 2 , 1 CaCl 2 , 10 HEPES, 11 EGTA and 2 adenosine triphosphate (pH 7.2). Cells were superfused with Krebs solution containing (mM): 140 NaCl, 4.7 KCl, 1.2 MgCl 2 , 2.5 CaCl 2 , 10 HEPES and 11 glucose (pH 7.4). Recordings were filtered at 5 kHz (6-pole Bessel, 36 dB per octave). Drugs and Krebs solution were applied using a modified U-tube. GABA, bicuculline, picrotoxin and ethanol were dissolved directly into Krebs solution (adjusted to pH 7.4). Allopregnanolone and diazepam were diluted in Krebs from a 10 mM stock in DMSO. For whole-cell studies of ethanol potentiation, the GABA current evoked by a low GABA concentration (EC 10 ) was initially determined, then 30–200 mM ethanol was applied for 30–60 s prior to the co-application of EC 10 GABA and ethanol. Allopregnanolone potentiation was determined by co-application with EC 10 GABA and the neurosteroid. Dose–response relationship data were fitted with a non-linear least squares fitting routine using Origin 6.1 (Microcal). Data points represent the mean ±s.e.m. of at least three experiments. The relative proportion of spontaneous GABA A receptor activation was ascertained by dividing the amplitude of currents induced by saturating concentrations of PTX ( I PTX ) by the summed current amplitudes induced by saturating concentrations of PTX and GABA ( I GABA + I PTX ). Single-channel currents were recorded at room temperature from excised outside-out membrane patches maintained at −70 mV (sampling rate 50 kHz; low pass-filtered at 10 kHz during recording, and at 2–5 kHz during analysis). Patches showing multiple simultaneous channel openings (channel stacking) exceeding 2% of all detected openings were discarded. Single-channel data were analysed using WinEDR (v.3.3.8; Strathclyde electrophysiology software, J Dempster) and QuB (2.0.0.13, Buffalo, NY). Amplitude histograms were created by fitting Gaussian components to the amplitude distributions using a non-linear least-squares routine. Open probabilities (Po) were defined as the ratio between the Gaussian areas of open and shut time components. Individual open and shut time durations were idealized using either WinEDR’s 50% threshold detection method or by QuB’s segmental k-means (SKM) fitting routine. Open and shut dwell-time histograms were fitted with a mixture of exponentials using a Levenberg–Marquardt non-linear least-squares method from which the areas representing the individual exponential components and their relative time constants were obtained. Mean dwell-time durations were calculated from the individual open and shut times weighted by their areas [33] , [46] , [47] . Confocal microscopy and immunocytochemistry GABA A R receptor α2, β1 myc or β1 myc,L285R or β1 myc,P228H , and γ2S or γ2L subunits were expressed with eGFP in HEK293 cells and incubated at room temperature with 9E10 antibody (to the extracellular myc epitope; Santa Cruz Biotechnology) followed by TRITC- or Cy5-conjugated secondary antibody. The myc epitope in the β1 subunit is electrophysiologically silent [48] . Transfected HEK293 cells were fixed in phosphate-buffered saline (PBS) containing 4% paraformaldehyde for 15 min before being quenched with 50 mM NH 4 Cl in PBS for 10 min. After washing in PBS, cells were incubated for 45 min at room temperature with 9E10 antibody. Cells were washed in PBS containing 10% v / v fetal calf serum (FCS) and 0.4% w / v bovine serum albumin (BSA) before incubation for 45 min with a TRITC- or Cy5-conjugated secondary antibody. Cells were washed and then mounted in glycerol before imaging using a Zeiss Axiophot confocal microscope (LSM510 Meta). The detector gain, and amplifier offset and gain were set at the same levels for all FITC, TRITC and Cy5 images of WT and mutant receptors to compare expression intensities. The scanning slice depth was set to 2.1 μm. Statistical analysis Analyses were performed using SPSS v14 and SigmaStat software (SPSS, USA). Data are presented as mean±s.e.m. or 95% confidence intervals unless otherwise stated. Student’s t -tests were used for two group comparisons (paired or unpaired as appropriate). Multifactorial linear model analysis was used to investigate the effect of genotype on alcohol preference, correcting for generation, gender and weight. Two-way ANOVA, with the between-subject factor ‘genotype’ and within-subject factor ‘session’, was used to evaluate potential genotype and reinforcer type effect and any interactions, and lever pressing in extinction. Categorized indices were compared using a Fisher’s exact test. The non-parametric Kolmogorov–Smirnoff test was used to compare cumulative probability distributions of IPSC parameters. Statistical significance was routinely set at P <0.05 and at P <0.01 for the Kolmogorov–Smirnoff test. How to cite this article: Anstee, Q. M. et al. Mutations in the Gabrb1 gene promote alcohol consumption through increased tonic inhibition. Nat. Commun. 4:2816 doi: 10.1038/ncomms3816 (2013).